Hyperlenses and metalenses for far-field super-resolution imaging Optical microscopy has revolutionized many fields such as microelectronics, biology and medicine. However, the resolution of a conventional optical lens system is always limited by diffraction to about half the wavelength of light. This diffraction barrier arises from the fact that subwavelength information from an object is carried by high spatial-frequency evanescent waves, which only exist in the near field. To overcome this diffraction limit, pioneering work has been carried out, including near-field scanning microscopy [1] , as well as fluorescence-based imaging methods [2] , [3] . These scanning- or random sampling-based non-projection techniques achieve super-resolving power by sacrificing imaging speed, making them uncompetitive for dynamic imaging. Lens-based projection imaging remains the best option for high-speed microscopy. Immersion techniques have been proposed to enhance resolution, but they are limited by the low refractive indices of natural materials [4] . Emerging within the last decade, the fields of plasmonics and metamaterials provide solutions for engineering extraordinary material properties not found in nature, such as negative index of refraction [5] , [6] or strongly anisotropic materials [7] , [8] . This has provided tremendous opportunities for novel lens designs with unprecedented resolution [9] . Initiated by Pendry’s seminal concept of the perfect lens [10] , a number of superlenses were demonstrated with resolving powers beyond the diffraction limit [11] , [12] , [13] , [14] , [15] , [16] , [17] . The optical superlens first achieved sub-diffraction-limited resolution by enhancing evanescent waves through a slab of silver [11] . As the evanescent-field enhancement is enabled by surface plasmon excitation, the subwavelength image is typically limited to the near field of the metal slab. However, the hyperlens—a metamaterial-based lens—can send super-resolution images into the far field by introducing a magnification mechanism. This has been considered as one of the most promising candidates for practical applications since its first demonstration in 2007 (refs 13 , 14 ). Recently, various other metamaterial-based lenses, that is, metalenses, have also been developed with both super-resolving power and Fourier transform function, making them more like conventional lenses but with superior capabilities [18] , [19] , [20] , [21] . In this review, we will describe the underlying physics of the hyperlens and metalens, their design principles, recent advances, major limitations and practical challenges, as well as suggestions for future development. The extension of the hyperlens concept from electromagnetic waves to acoustic waves is also included. In addition, we will discuss some of the other super-resolution techniques, such as near-field scattering and the time-reversal technique. Light emission or scattering from objects comprises both propagating and evanescent components, corresponding to low and high wave-vectors, respectively. The propagating waves carrying large-feature information reach the far field, whereas the evanescent waves containing the detailed information are non-propagating in a normal material environment, and are thus confined to the near field. Diffraction-limited imaging originates from the fact that the deep subwavelength information carried by the evanescent waves cannot reach the far field and so does not contribute to the formation of the final image. The realization of the hyperlens for far-field super-resolution imaging relies on two basic requirements: a material that supports wave propagation with high wave-vectors; and a magnification mechanism, that is, conversion of high wave-vector waves to low wave-vector waves so that the super-resolution information can be sent to the far field. Anisotropic plasmonic metamaterials provide one of the most practical options to fulfil the material requirement, for which there is no need to deal with the design of permeabilities but only permittivities along different directions; thus, the overall material loss is significantly reduced [8] , [22] . The simplest anisotropic plasmonic metamaterials can be constructed by the deposition of alternating metal/dielectric multilayers ( Box 1 ). When the layer thickness is much smaller than the probing wavelength, an effective-medium approximation is commonly used to describe the permittivities along different directions, that is, ɛ x , ɛ y and ɛ z (ref. 23 ). Although the term ‘hyperlens’ was applied to metamaterials with a hyperbolic dispersion relationship, that is, ɛ x = ɛ y and ɛ z taking different signs [15] , elliptically dispersive metamaterials can also be used to build a hyperlens as long as the coverage for lateral wave-vectors is large enough [24] . The magnification mechanism, that is, the wave-vector compression, is obtained by bending the flat layers into co-centrically curved layers [9] , [15] , which can be explained through transformation optics [25] . Owing to the conservation of angular momentum, the tangential wave-vectors are progressively compressed as the waves travel along the radial direction. A magnified image carried by low wave-vectors will ultimately be formed at the outer boundary of the hyperlens before propagating into the far field, supported by the surrounding environment. The magnification at the output surface is given simply by the ratio of the radii at the two boundaries. Practical configurations of the hyperlens were proposed by different groups, including a cylindrical geometry [15] , [25] , [26] , tapered metallic wire arrays [27] , [28] , [29] , [30] or uniquely designed material dispersions [31] , [32] , [33] , [34] . To circumvent the problem of absorption in real materials and thereby avoid image distortions in the far field, proper configurational design must ensure that all rays originating from the object plane travel equal path lengths through the metamaterial. Scattering at surfaces of the hyperlens, however, has proven detrimental for real imaging applications. Design rules have been proposed to impedance match the hyperlens metamaterial with both inner and outer boundaries using radius-dependent magnetic permeability [35] . Comparable performance through the reduction of surface reflections can be achieved in non-magnetic metamaterials by impedance matching at one of the hyperlens surfaces instead of both. This trade-off has been confirmed by simulations and can be practically implemented [35] , [36] . Owing to its use of curved surfaces, the cylindrical hyperlens design may not be convenient for bio-imaging. Design of the planar hyperlens has been shown to be theoretically feasible via specific material dispersion based on transformation optics [31] , [32] , [37] . In such designs, the metamaterial properties are designed to bend light rays from subwavelength features in such a way as to form a resolvable image on a flat output plane. Box 1: Hyperlens and anisotropic metamaterials. Coarse and fine information from objects, corresponding to low and high wave-vector components, is carried by propagating and evanescent waves, respectively. Only propagating waves can reach the far field to be collected by a lens system, leading to the so-called ‘diffraction limit’. Unlike isotropic media with a spherical dispersion, the dispersion properties for multilayer metamaterials can be designed to have for hyperbolic dispersions or for eccentric elliptic dispersions, where represent the real part of the permittivity along x and z directions (top left). Anisotropic metamaterials support the propagation of high wave-vector waves due to their unbounded wave-vector values or very large wave-vector cutoff. By using different material combinations, the working wavelength for multilayered metamaterials can be tuned across a broad band of wavelengths. Metallic nanowire-based metamaterials can also be used but cause shifts towards much longer operational wavelengths. The wavelength range for either hyperbolic or elliptic dispersion is determined by not only the constituents’ permittivity but also their filling ratios. Anisotropic multilayer metamaterials in a curved geometry result in hyperlenses with corresponding dispersions represented in cylindrical coordinates (top right). For a subwavelength object placed at the inner boundary, wave propagation along the radial direction gradually compresses its tangential wave-vectors, resulting in a magnified image at the outer boundary. The magnified image, once larger than the diffraction limit, will be resolved in the far field. The bottom row shows that two sub-diffraction-limited line sources separated by a distance of ∼ 80 nm can be clearly resolved by using either eccentric elliptic (left) or hyperbolic (middle) metamaterials, but not by air alone (right). In the simulation, the radii of the hyperlens of either dispersion at the inner and outer boundaries are ρ inner =240 nm and ρ outer =1,200 nm, respectively. The permittivity for metal and dielectric in the hyperbolic (elliptic) hyperlens is −2.3–0.3i (−2.3–0.3i) and 2.7 (2.25), respectively. The filling ratio of metal in both hyperlenses is 50%. Theoretical predictions about hyperlenses, using anisotropic media composed of curved multilayer stacks [15] , [26] , have inspired experimental investigations into the hyperlens concept. The first one-dimensional (1D) optical hyperlens was demonstrated at ultraviolet frequencies by conformal deposition of Ag and Al 2 O 3 multilayer films on a cylindrical quartz cavity ( Fig. 1a ) [13] , [38] . A sub-diffraction-limited object with a 130-nm centre-to-centre distance was observed directly in the far field ( Fig. 1b ). The magnified hyperlens image shows the object clearly resolved, as compared with a diffraction-limited image in a control experiment. So far, hyperlens experiments have achieved 125 nm-pitch resolution (λ/2.92) working at a wavelength of 365 nm (ref. 38 ), although some simulations provided designs with much higher resolution around λ/9 (ref. 39 ). A different approach to realizing cylindrical magnifying superlenses uses surface plasmon waves confined on a metal surface with a concentric polymer grating [14] . The magnified images of the surface waves after scattering by the surface roughness were collected by a microscope. 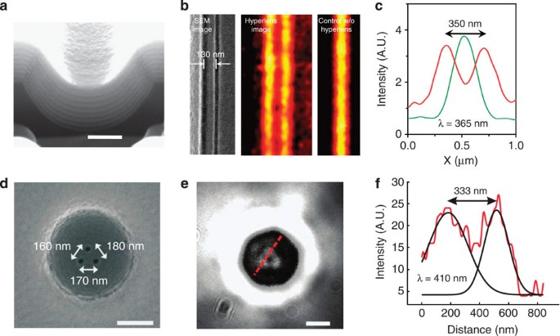Figure 1: Experimental demonstration of the optical hyperlens. (a) Scanning electron microscope (SEM) image of the cross section of a cylindrical hyperlens structure with 16 Ag (bright) and Al2O3(dark) layers. Reproduced with permission from ref.38. The thick bright layer at the top is chromium. All scale bars shown in the figure are 500 nm. (b) Hyperlens imaging of a pair of line objects with a line width of 35 nm and a centre-to-centre distance of 130 nm. From left to right, SEM image of the line-pair object, magnified hyperlens image, and the resulting diffraction-limited image in a control experiment. (c) The cross-section profile for the hyperlens image of the line-pair object (red) and for a diffraction-limited image obtained without the hyperlens (green). A.U., arbitrary units. (b,c) From ref.13(reproduced with permission from AAAS). (d) SEM image of three dots positioned triangularly with gaps of 180, 170 and 160 nm on a spherical hyperlens comprises nine pairs of Ag and Ti3O5layers. (e,f) Image of the object after being magnified and its cross section along the red dashed line. The black curves in (f) correspond to the cross-sectional analysis for identifying the separation of the two apertures measured to be 333 nm. (d–f), From ref.17. Figure 1: Experimental demonstration of the optical hyperlens. ( a ) Scanning electron microscope (SEM) image of the cross section of a cylindrical hyperlens structure with 16 Ag (bright) and Al 2 O 3 (dark) layers. Reproduced with permission from ref. 38 . The thick bright layer at the top is chromium. All scale bars shown in the figure are 500 nm. ( b ) Hyperlens imaging of a pair of line objects with a line width of 35 nm and a centre-to-centre distance of 130 nm. From left to right, SEM image of the line-pair object, magnified hyperlens image, and the resulting diffraction-limited image in a control experiment. ( c ) The cross-section profile for the hyperlens image of the line-pair object (red) and for a diffraction-limited image obtained without the hyperlens (green). A.U., arbitrary units. ( b , c ) From ref. 13 (reproduced with permission from AAAS). ( d ) SEM image of three dots positioned triangularly with gaps of 180, 170 and 160 nm on a spherical hyperlens comprises nine pairs of Ag and Ti 3 O 5 layers. ( e , f ) Image of the object after being magnified and its cross section along the red dashed line. The black curves in ( f ) correspond to the cross-sectional analysis for identifying the separation of the two apertures measured to be 333 nm. ( d – f ), From ref. 17 . Full size image The cylindrical hyperlens only provides 1D resolution improvement, which limits its use in practical applications. A spherical hyperlens with two-dimensional (2D) super-resolution capability is far more desirable, and has recently been experimentally demonstrated for the visible spectral region [17] . This 2D hyperlens was created by deposition of alternating layers of Ag and Ti 3 O 5 thin films in a hemispherical geometry designed with a hyperbolic dispersion that supports the propagation of very high spatial-frequency waves at the same phase speed. An object with spacing down to 160 nm in a triangular configuration on the spherical hyperlens ( Fig. 1d ) is clearly resolved in the far field ( Fig. 1e ), beyond the diffraction limit, 205 nm, at a wavelength of 410 nm. The corresponding separation of the image is measured to be 333 nm in the cross-sectional analysis shown in Fig. 1f , resulting in an averaged magnification factor of 2.08. These proof-of-concept experiments have produced hyperlenses with hyperbolic dispersions working at ultraviolet and visible wavelengths. With appropriate material combinations, a broad working range across the visible or near-infrared becomes attainable for both hyperbolic dispersions and highly elliptical dispersions [36] . The resolution of hyperlenses is essentially determined by the geometry, material loss and also the film quality. In addition to increasing the magnification with a higher ratio of the outer-to-inner radii, the resolution could be further improved through the choice of appropriate filling ratios of metal and dielectric components because, as the dispersion approaches flatness, it results in the transport of even higher spatial-frequency information [36] . Although the intrinsic metal loss is unavoidable, the hyperlens can be optimized by increasing the amount of the dielectric component or working at longer wavelengths. A higher optical transmission can also be realized with resonant structures [40] , [41] . Moreover, instead of conformal film deposition, fabrication based on rolled-up technology provides an alternative method for controlling film conformality and roughness [41] , [42] , [43] , [44] . Another super-resolution scheme based on metallic wire arrays was proposed to attain a wide range of working wavelengths over a long transport distance [27] . Experimental demonstrations, however, were limited to subwavelength imaging in the near field using metallic wires grown in dielectric templates [45] , [46] . The tapered nanorod array with a magnification mechanism for far-field imaging still suffers critical challenges in achieving accurate growth at tapered angles and introducing gaps between the arrays [47] . With increased efforts towards the development of growth technologies [48] , [49] , [50] , experimental demonstrations of the proposed scheme for subwavelength colour imaging could become a reality in the near future. The hyperlens discussed so far, although capable of super-resolution for far-field detection, lacks the ability to focus plane waves. For conventional optical lenses, refraction and focusing of light rely on curved interfaces, fundamental for Fourier transforms and imaging. However, hyperlenses cannot realize the Fourier transform function due to their lack of a phase compensation mechanism. In this and the following sections, we will introduce the metalens: a metamaterial-based lens that provides not only the advantages of super-resolving capabilities but also the Fourier transform function, making it an exceptional combination of super-resolution and desirable functions of conventional lenses. A metalens is created by combining a metamaterial slab and a phase compensation mechanism to bring a plane wave to a focus ( Box 2 ). Anisotropic metamaterials with either a hyperbolic or eccentric elliptic dispersion are essential for supporting the propagation of super-resolution information carried by high wave-vectors. The hyperlens and the metalens thus share the same material requirement, with practical realizations including multilayers [13] and nanowire metamaterials [22] . On the other hand, as high wave-vector waves are totally reflected at the metamaterial–air interface, a bidirectional coupler is needed to convert waves from high wave-vectors in the metamaterial to low wave-vectors in air, and vice versa. To make a focusing lens, this coupler must also function as a phase compensation mechanism, in contrast with the far-field superlens that functions as an evanescent-to-propagating convertor through the use of a grating [16] . Various types of phase compensation mechanism have been proposed for focusing plane waves in metalenses [18] , [19] , [20] . The underlying design principle is to satisfy the phase matching condition to constructively bring plane waves from air into deep subwavelength focus inside the metamaterial. This can be accomplished by either geometric variations, such as plasmonic waveguide couplers (PWC) [18] , [51] , [52] , [53] and shaped metamaterial–air interfaces [19] , [54] , or material refractive-index variations like gradient-index (GRIN) metamaterials [20] . For example, a PWC, composed of an array of specially designed non-periodic metal-insulator-metal waveguides, can turn non-flat wave-fronts at the metamaterial–PWC interface into flat ones at the PWC–air interface, thus matching the phase condition for realizing a deep subwavelength focus inside the metamaterial slab [18] , [51] . Instead of relying on metal-insulator-metal waveguides, a metamaterial with a hyperbolic dispersion can also achieve low and high wave-vector conversion and phase compensation after being shaped to a concave surface. In contrast, a convex surface is needed for metamaterials with an elliptic dispersion. The curvature of the metalens is determined by a lens maker’s equation that is similar to the conventional one [19] . Using transformation optics [55] , [56] , such geometry variations can be transformed to refractive-index variations within the material space, resulting in a GRIN metalens. Analogous to a conventional GRIN lens [57] , the designed permittivity profiles for a GRIN metalens gradually bring plane waves to a super-resolution focus inside the metamaterial [20] , [58] . Box 2: Principle of the metalens. The essence of a lens is to modify the phase of an incident plane wave to form a focus. There are generally three methods to introduce a phase compensation mechanism into a lens design: shaping the surface of a piece of homogenous material, such as polishing a piece of glass to have a convex surface; use of diffractive structures to engineer the wavefront, as is done with the Fresnel zone plate; using material inhomogeneity to modify the phase change in space with, for instance, a GRIN lens. The metalens applies similar phase compensation mechanisms to metamaterials to bring a plane-wave to a focus. To achieve practical sub-diffraction-limited resolution, the metamaterials have to satisfy the same material requirements as those for a hyperlens. As high spatial-frequency waves inside a metamaterial cannot transmit to air due to total internal reflection, a bidirectional coupling mechanism is needed to convert waves from high spatial frequency in the metamaterial to low spatial frequency in air, or vice versa. Analogous to conventional lenses, various coupling schemes can fulfil this task, including metamaterials with shaped interfaces (left), a planar plasmonic metal-insulator-metal waveguide coupler (middle) and GRIN metamaterials (right). When the focal length is defined, the imaging magnification is obtained by placing an object at an appropriate distance from the metalens, which is similar to the case of a conventional lens. One demonstration of the metalens was first proposed by utilizing a planar PWC at ultraviolet wavelengths [18] . Based on a silver PWC, the metalens with an elliptic dispersion achieved a deep subwavelength focal spot with a full width at half maximum of 59 nm ( ∼ λ/6.2) in the metamaterial [18] . Compared with the diffraction-limited focal spot in air, about threefold resolution improvement was demonstrated. A similar improvement for a hyperbolic metalens based on a planar aluminium PWC is also possible [18] . Under the same design principle, an alternative PWC satisfies the phase condition by tuning the waveguide height instead of width. Improved resolution ( ∼ λ/8.6) was verified at longer wavelengths, due to smaller material loss [51] . Although the PWC-based metalens is capable of exceptional imaging resolution, it may demand a sophisticated fabrication process. As a metamaterial counterpart to the solid immersion lens [4] , [59] , metalenses formed by shaping metamaterial surfaces have recently been proposed for super-resolution imaging with the Fourier transform function [19] . Using a convex geometry, an elliptic metamaterial made of multilayers of silver and gallium phosphide can satisfy the phase compensation condition for subwavelength focusing. A deep subwavelength focal spot with a full width at half maximum of 70 nm ( ∼ λ/9) was formed at a focal length of 3 μm for normal plane-wave incidence at a red wavelength of 633 nm (ref. 19 ). This metalens achieved an effective numerical aperture of 4.5, which is much larger than that found in naturally occurring materials [60] , [61] . In addition, owing to negative refraction, a hyperbolic metamaterial must be made into a concave geometry to focus light, which is exceptionally different from the requirement for conventional lenses [19] . Such geometry manipulation can alternatively be converted to spatially variant material property design. Inhomogeneous metamaterials have been utilized to focus light in the infrared [58] , [62] or surface waves [63] . The GRIN metalens, with appropriately designed permittivity profiles, was first investigated for its super-resolution imaging, as well as its Fourier transform capabilities at optical wavelengths [20] . The hyperbolic permittivity profile, enabled by the use of silver nanowires grown in an alumina template, gradually converges a normally incident wave to a sub-diffraction-limited focus inside the metamaterial ( Fig. 2 ). When the metalens is truncated at a plane close to the internal focus, the super-resolution focus on the truncated surface can be accessed externally ( Fig. 2 ). 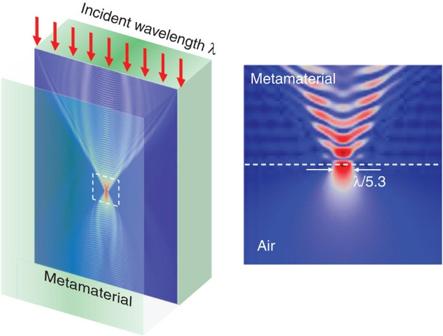Figure 2: Numerical demonstration of a GRIN metalens. A hyperbolic GRIN metalens forms a sub-diffraction-limited internal focus inside the metamaterial. A full width at half maximum of 156 nm (λ/5.3) is obtained at the illumination wavelength of λ=830 nm when the lens is truncated at the focal plane, as shown on the right, which displays a zoom-in of the boxed region around the focus. Reproduced, with permission, from ref.20. Copyright 2011 by the American Physical Society. Figure 2: Numerical demonstration of a GRIN metalens. A hyperbolic GRIN metalens forms a sub-diffraction-limited internal focus inside the metamaterial. A full width at half maximum of 156 nm (λ/5.3) is obtained at the illumination wavelength of λ=830 nm when the lens is truncated at the focal plane, as shown on the right, which displays a zoom-in of the boxed region around the focus. Reproduced, with permission, from ref. 20 . Copyright 2011 by the American Physical Society. Full size image All the metalenses introduced above were built based on real material properties. In addition to material and coupling loss, non-monochromatic illumination may reduce the focusing performance, as the metamaterials are made of dispersive metal and dielectric composites. Nonetheless, they work fairly well in a relatively wide range of wavelengths, and can always be optimized for further resolution improvement by careful choice of material combinations for desired working wavelengths. Here, we mainly focused on super-resolution focusing in 1D at optical frequencies. Yet these principles can be easily extended to 2D, as well as to other frequencies, such as the infrared, terahertz, or microwave regions. The same principles can also be applied to acoustics due to the nature of waves. The metalens exhibits deep subwavelength plane-wave focusing with a defined focal length, which is in stark contrast to the hyperlens. The imaging properties of a lens, that is, the image characteristics of an object placed at different locations with respect to the lens focal length f , are well understood, being governed by the imaging equation 1/ s o +1/ s i =1/ f , where s o and s i are the object and image distances to the lens, respectively. A metalens achieves subwavelength focusing by combining either hyperbolic or elliptically dispersive metamaterials with a phase compensation mechanism. Notice that the hyperbolic metalens has negative refraction at the metalens-air interface, leading to an opposite focal shift with respect to the tilted incident plane waves [18] , [19] , [20] . Unprecedented imaging properties are expected from such lenses with abnormal Fourier transform properties [21] . Consider a PWC-based hyperbolic metalens that comprises a PWC and a metamaterial slab with hyperbolic dispersion . A plane wave incident from the air side converges to the focus F m at a focal length of f m in the hyperbolic metamaterial side ( Fig. 3a ). Meanwhile, a plane wave from the metamaterial side diverges after passing through the metalens, resulting in a virtual focus at F d at a focal length of f d also in the metamaterial ( Fig. 3b ). In contrast to a converging lens with one focus on either side, this distinctive focusing behaviour makes the hyperbolic metalens into a ‘Janus lens’, having two different focusing behaviours in opposite directions. 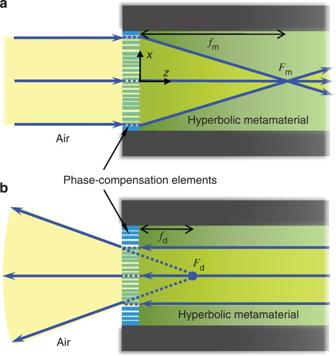Figure 3: Extraordinary focusing property of a Janus lens. (a) Plane waves from air converge through a phase-compensating element to a focus (Fm) in the metamaterial. (b) Plane waves from the metamaterial diverge in air, resulting in a virtual focus (Fd) also in the metamaterial. The arrows in (a) and (b) are eye-guiding rays. Figure 3: Extraordinary focusing property of a Janus lens. ( a ) Plane waves from air converge through a phase-compensating element to a focus ( F m ) in the metamaterial. ( b ) Plane waves from the metamaterial diverge in air, resulting in a virtual focus ( F d ) also in the metamaterial. The arrows in ( a ) and ( b ) are eye-guiding rays. Full size image For a Janus lens, the imaging behaviour is governed by a new metalens imaging equation [21] , or where v d and v m are the image and object distances in air and metamaterial, respectively; the focal lengths satisfy . In contrast to the conventional imaging equations, the material properties for a metalens also have an important role in its imaging characteristics. Therefore, the Janus-lens imaging properties with respect to the focal lengths are completely different from those of a conventional glass lens [64] . For example, the Janus-lens image of an object in air is always minified, erect and real within the first focal length inside the metamaterial. In contrast, a glass lens image may be magnified, erect and imaginary if it is too close to the lens, as in the case for a magnifying lens. When the metalens is truncated to a plane within F m , a magnified real image is formed in air for a subwavelength object placed on the truncated surface of the metamaterial [21] . Therefore, a super-resolution image for far-field detection becomes possible. Hyperbolic metalenses having this type of new imaging property, in addition to super-resolution, pave the way for novel optical devices and systems that could be extremely hard to achieve with conventional lenses. Both hyperlenses and metalenses achieve super-resolution imaging with the use of anisotropic metamaterials that support the propagation of high spatial-frequency waves and a magnification mechanism for detection in the far field. Alternative approaches have been proposed for sub-diffraction-limited imaging utilizing inversion procedures with far-field detection, including time reversal, optical diffraction tomography (ODT) and compressed sensing [65] , [66] , [67] , [68] , [69] , [70] . The time-reversal technique was first introduced as an inversion method for electromagnetic waves and was experimentally demonstrated by subwavelength focusing and imaging of microwaves [65] , [66] , [71] , [72] , [73] , [74] , [75] . Evanescent waves that carry small details are converted into propagating waves by placing a subwavelength object made of monopoles in the near field of a cluster of strongly coupled resonators, referred to as a ‘resonant metalens’ ( Fig. 4 ). In contrast to the metalens that uses a narrow band of frequencies, the resonant metalens takes advantage of the strong dispersive properties of the resonator structures. The broadband emission from the object generates a subwavelength profile at the input of the lens. Coupling between the source and the eigenmodes inside the resonant metalens efficiently scatters off near-field information, which is encoded in time and recorded by far-field antennas in different directions ( Fig. 4 ). Using time reversal, the far-field detection is ‘flipped’ in time and reemitted from the same antenna locations. The time-reversed signal arrives at the lens and is recorded by the monopoles, now acting as receivers. Based on the reciprocity of the system, not only propagating waves but also evanescent waves can be recovered at the monopole location. An image with a sub-diffraction-limited resolution of λ/80 has been reconstructed by cross-correlation between the received signals and the filters [66] , [72] . An extension to 2D imaging is possible by using a total internal reflection configuration [72] . The resolution of such a resonant metalens is affected by the period of the wires, as well as the loss in metals, which cannot be compensated by time reversal. It may be possible to extend this proof-of-concept from the microwave range to the near-infrared or visible, although the details of resonator design and experimental methodology may be very different [76] , [77] . 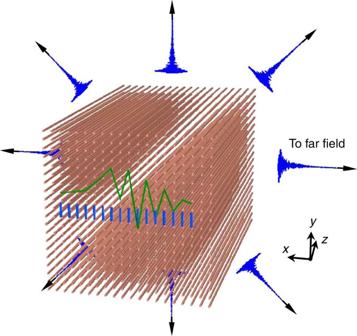Figure 4: Super-resolution based on time reversal. Schematic configuration of a resonant metalens made of an array of copper wires with a subwavelength period of about λ/80 placed on the ground on top of a copper plate (the copper plate has been removed for clarity). A subwavelength object consisting of 16 small monopoles with a period of λ/80 (blue line array) is placed between the ground plane and the metalens. The emission amplitude profile of the array is shown in green (data from ref.66). Time-resolved signals scattered off the metalens propagate into the far field to be collected by far-field antennas in different directions. Figure 4: Super-resolution based on time reversal. Schematic configuration of a resonant metalens made of an array of copper wires with a subwavelength period of about λ/80 placed on the ground on top of a copper plate (the copper plate has been removed for clarity). A subwavelength object consisting of 16 small monopoles with a period of λ/80 (blue line array) is placed between the ground plane and the metalens. The emission amplitude profile of the array is shown in green (data from ref. 66 ). Time-resolved signals scattered off the metalens propagate into the far field to be collected by far-field antennas in different directions. Full size image In contrast to the inversion procedure based on temporal signal reversal, another approach, widely known as ODT or synthetic aperture digital holography, reconstructs the image using multiple measurements of both the amplitude and phase of the field diffracted by an unknown object at many incident angles [78] , [79] , [80] . Recently, it has been studied with the goal of breaking the diffraction limit in far-field optical imaging [67] , [68] , [81] , [82] , [83] . The resolution is improved by measurements at many incident angles that enlarge the accessible range of spatial frequencies. The permittivity or shape, intrinsic properties of the object, are then reconstructed numerically by well-developed inversion algorithms that iteratively minimize the discrepancy between the measured scatter field and that simulated via a forward solver [68] . The resolution performance of ODT depends on various factors, including the number of incidences and observation points, covered angular range, inversion algorithms, and system noise level. Although a moderate resolution improvement has been demonstrated experimentally [68] , the imaging speed is limited by the need for multiple measurements. As in the case for electromagnetic waves, the resolution for conventional acoustic imaging is also limited by the wavelength of acoustic waves due to loss of spatial details carried by evanescent waves. The concept of anisotropic metamaterials has therefore been suggested for super-resolution imaging of acoustic waves for potential applications in sonar sensing, ultrasonic imaging and non-destructive material testing [84] , [85] , [86] . In 2009, a 2D acoustic hyperlens was experimentally demonstrated for deep-subwavelength imaging over a broadband frequency range and with low loss [87] . It consists of a non-resonant radially symmetric layered structure similar to the optical hyperlens, but with tapered metallic wires that gradually convert evanescent waves into propagating waves in the far field ( Fig. 5 ). Two sound sources with a subwavelength separation of 1.2 cm were well resolved at the outer surface of the hyperlens when the frequency was swept from 4.2 to 7 kHz, corresponding to a λ/6.8 to λ/4.1 resolution. Owing to their longitudinal nature, the dispersion relation for acoustic waves is described by the effective mass density together with the effective bulk modulus [88] . Instead of using a hyperbolic dispersion, the acoustic hyperlens has a highly eccentric elliptic dispersion with positive effective mass density that supports a broadband working frequency and a large range of wave-vectors. With an elliptic rather than a hyperbolic dispersion, it avoids the use of resonating elements in constructing the metamaterial, resulting in a low-loss hyperlens with very large propagation distances and, thus, a very large magnification. This kind of anisotropic acoustic metamaterial was later utilized in the fabrication of a 3D holey-structured metamaterial for acoustic deep-subwavelength imaging [89] . A 2D object with a line width of 3.18 mm can be clearly resolved at the operating frequency of 2.18 kHz, demonstrating a subwavelength resolution of λ/50 (ref. 89 ). This was achieved by the effective transmission of evanescent wave components carrying deep-subwavelength details to the output side through the Fabry–Pérot resonances excited inside the holey structure. Although the nearly perfect imaging was confined to the near field of the acoustic metamaterial, it points to a possibility for constructing a 3D hyperlens for far-field subwavelength imaging by perforating a hemispherical solid with tapered holes in the radial direction. In addition to deep subwavelength imaging, other applications of acoustic metamaterials for extreme manipulation of acoustic waves include focusing, cloaking and extraordinary transmission or absorption [90] , [91] , [92] , [93] . 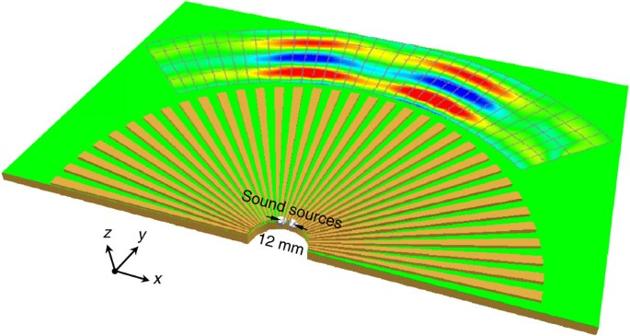Figure 5: Super-resolution imaging of acoustic waves. A 2D acoustic hyperlens made of 36 brass fins (running radially from a radius of 2.7–21.8 cm) in air embedded on a brass substrate, spanning 180° in the angular direction. The cover aluminium sheet has been removed to expose the microstructure for this view. The intensity profile in the green background represents experimental pressure measurements from ref.87in the propagation region that show a magnified image of a sub-diffraction-limited object consisting of two in-phase sound sources separated by 1.2 cm at 6.6 kHz. The pressure is measured at various points ranging from 0.4 to 9.9 cm away from the lens. Figure 5: Super-resolution imaging of acoustic waves. A 2D acoustic hyperlens made of 36 brass fins (running radially from a radius of 2.7–21.8 cm) in air embedded on a brass substrate, spanning 180° in the angular direction. The cover aluminium sheet has been removed to expose the microstructure for this view. The intensity profile in the green background represents experimental pressure measurements from ref. 87 in the propagation region that show a magnified image of a sub-diffraction-limited object consisting of two in-phase sound sources separated by 1.2 cm at 6.6 kHz. The pressure is measured at various points ranging from 0.4 to 9.9 cm away from the lens. Full size image Despite all the success achieved by acoustic metamaterials, other strategies such as time-reversal techniques [94] , [95] have also been extended to overcome acoustic imaging limitations. Based on a sonic analogue to the resonant metalens proposed for electromagnetic waves [65] , [66] , one group recently proved by experiment that broadband sounds can be controlled and focused on a subwavelength scale by using acoustic resonators [94] . The demonstration of foci with a λ/25 size for audible sound testifies to the generality of the time-reversal principle. Nevertheless, experimental proof of the capability of the time-reversal metalens for subwavelength imaging is still needed. Over the past few years, the hyperlens, relying on anisotropic metamaterials with magnifying power, has been demonstrated to achieve sub-diffraction-limited resolution for far-field detection across the optical regime. On the other hand, the metalens has recently been proposed as a new member of the superlens family, having not only super-resolution power but also Fourier transform function due to the incorporation of a phase compensation mechanism, which makes it a more suitable candidate for integration with conventional optical systems. Although theoretical analysis and numerical simulations have proven its deep subwavelength focusing performance, as well as extraordinary imaging properties as a Janus lens, experimental demonstration of the metalens is necessary to prove its practical feasibility. In addition, there seem no physics limitations for the demonstration of the time-reversal imaging technique at optical frequencies, but necessary experimental technologies need to be developed before the technique can be effectively implemented. The possibilities for combining the time-reversal technique with hyperlenses or metalenses may yet become an interesting field worth exploring. There are two major limitations to future applications of both hyperlenses and metalenses. First, material loss is an intrinsic property of metamaterials at optical wavelengths, limiting the ultimate resolution of the lens, as well as the signal transmission efficiency, especially when resonant elements are involved. To mitigate the loss problem, several approaches may provide solutions, such as compensating for loss in the metal by addition of a gain medium in dielectrics [96] , searching for better plasmonic materials among existing elements, band structure engineering or materials doping or alloying [97] , [98] . Second, the object has to be placed in the near field of the lens to make use of the evanescent waves that normally decay away from the object, although the image can be projected and detected in the far field. This is also true for super-resolution imaging based on time-reversal and ODT. Super-resolution is thus limited to surface imaging, which may encounter difficulties in extension to the third dimension. New imaging schemes may be needed to solve this issue. Besides, current designs for both hyperlenses and metalenses have very limited field of view due to the limited physical size of the lens. Better designs, such as periodic array geometries with improved field of view to lens-diameter ratio, may solve the problem but it remains wide open to solutions. Image distortion and corresponding compensation methods are also important issues that need further investigations for practical applications of these lenses. In the case of hyperlenses, imaging at the back focal plane may result in a great reduction in distortions. Despite existing limitations, super-resolution with hyperlenses and metalenses has already shown exciting potential applications in various fields of science and technology. The implementation of these lenses in conventional optical microscopes may extend the resolution to the nanometre scale for real-time observations, which would have a great impact on modern biological imaging. Further improvement is expected by combining hyperlenses or metalenses with other imaging techniques, such as dark-field microscopy for high contrast microscopy [99] . Super-resolution imaging and its reversed process for writing may find applications in optical lithography and ultrahigh-density optical data storage [39] . The extension of the hyperlens and metalens concept to acoustic waves will also lead to super-resolution in applications such as sonar sensing and ultrasonic imaging. How to cite this article: Lu, D. et al . Hyperlenses and metalenses for far-field super-resolution imaging. Nat. Commun. 3:1205 doi: 10.1038/ncomms2176 (2012).